Nanostructural hierarchy increases the strength of aluminium alloys Increasing the strength of metallic alloys while maintaining formability is an interesting challenge for enabling new generations of lightweight structures and technologies. In this paper, we engineer aluminium alloys to contain a hierarchy of nanostructures and possess mechanical properties that expand known performance boundaries—an aerospace-grade 7075 alloy exhibits a yield strength and uniform elongation approaching 1 GPa and 5%, respectively. The nanostructural architecture was observed using novel high-resolution microscopy techniques and comprises a solid solution, free of precipitation, featuring (i) a high density of dislocations, (ii) subnanometre intragranular solute clusters, (iii) two geometries of nanometre-scale intergranular solute structures and (iv) grain sizes tens of nanometres in diameter. Our results demonstrate that this novel architecture offers a design pathway towards a new generation of super-strong materials with new regimes of property-performance space. Nearly 30 years passed between the discovery of the age-hardening effect by Alfred Wilm in 1906 and the X-ray scattering observations that established the link between this effect and the alloy microstructure [1] , [2] , [3] . It was yet another 20 years before more sensitive X-ray techniques and transmission electron microscopy (TEM) revealed more detailed microstructural origins and correlated age hardening to clusters of solute atoms and precipitate particles [4] , [5] . In the decades to follow, optimization of the type, size and dispersion of these microstructural features has produced sophisticated alloys now relied upon in many technologies [6] . Such a discovery into structure-to-property origins is a good example of how advances in characterization techniques and instrumentation can enable breakthroughs in materials science and engineering. Age-hardening effects are now widely used in modern aerospace, automotive and construction materials. In age-hardened aluminium (Al) alloys, relatively high yield strengths, ≥0.5 GPa, are achieved from thermomechanical treatments that generate precipitation-strengthened microstructures. Significantly, these microstructures retain reasonable (>5%) levels of uniform elongation in accordance with requirements for structural engineering applications. A survey of property-performance space for a wide range of metallic Al alloys indicates that values of yield strength of ~0.7 GPa represent the upper strength limit for precipitation-strengthened wrought Al alloys [6] , [7] , [8] , [9] . Severe plastic deformation (SPD) techniques emerged in 1991 as a novel processing strategy to effect grain refinement strengthening with potential for significant property enhancements [10] , [11] . In the 18 years leading up to the present, SPD alloys have attracted substantial interest, both for fundamental research and technological development [8] , [9] , [11] , [12] , [13] , [14] , [15] , [16] , [17] , [18] . It is now possible, through a variety of SPD techniques, to produce essentially homogenous microstructures exhibiting nanoscale grain refinement, provided select processing pathways are chosen and sufficiently high strain is imparted [14] , [19] , [20] . 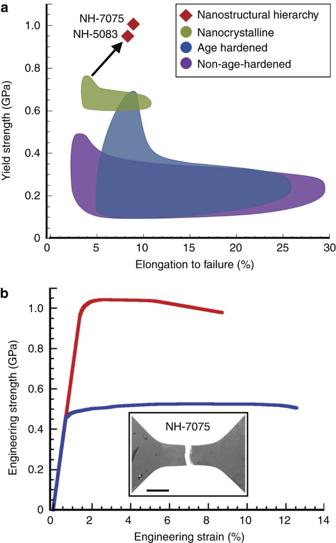Figure 1: Mechanical property performance of aluminium alloys. Two new aluminium alloys exhibiting record properties and solute nanostructure hierarchies (NH-7075, NH-5083). (a) A summary of the tensile properties of metallic Al alloys based on experimental data6,7,8,9,11,12,13,14,15,16,17,18. (b) A typical engineering stress–strain plot for the NH-7075 (red curve) and T6-7075 (blue curve) alloys indicates that the HPT processing achieves nearly twice the strength of the highly used and commercially valuable T6 treated alloy. Inset is the fractured tensile specimen of the NH-7075 Al alloy; scale bar, 1 mm. Apart from a record breaking yield strength of nearly 1 GPa, it is significant that the NH-7075 alloy exhibits a uniform elongation of ~5%, and total elongation-to-failure is as high as 9%. As seen in Figure 1a , Al alloys produced by SPD have recently exhibited tensile yield strengths as high as ~0.75 GPa and elongations up to ~10% [8] , [9] . Such SPD alloys are typically strengthened by refined grain dimensions, as well as by the propensity for high dislocation accumulation and by precipitate particles. Figure 1: Mechanical property performance of aluminium alloys. Two new aluminium alloys exhibiting record properties and solute nanostructure hierarchies (NH-7075, NH-5083). ( a ) A summary of the tensile properties of metallic Al alloys based on experimental data [6] , [7] , [8] , [9] , [11] , [12] , [13] , [14] , [15] , [16] , [17] , [18] . ( b ) A typical engineering stress–strain plot for the NH-7075 (red curve) and T6-7075 (blue curve) alloys indicates that the HPT processing achieves nearly twice the strength of the highly used and commercially valuable T6 treated alloy. Inset is the fractured tensile specimen of the NH-7075 Al alloy; scale bar, 1 mm. Apart from a record breaking yield strength of nearly 1 GPa, it is significant that the NH-7075 alloy exhibits a uniform elongation of ~5%, and total elongation-to-failure is as high as 9%. Full size image There remains an unsatisfactory fit between theory-based structure–property relationships in SPD metals. For example, the veracity of Hall–Petch-type relationships as the grain size reduces below 100 nm is problematic [21] , [22] , [23] . Anomalies in grain coarsening phenomena have been widely reported, and there is much uncertainty about the precise deformation modes [24] , [25] , [26] . This suggests strongly that new experimentally derived insights into the nanostructure are needed to comprehensively describe the structures within these unusual materials and their influences on properties. Here, it must be noted that electron microscopy and microanalysis of such nanoscale grains is particularly challenging. Images from the thinnest foils in TEM contain convolutions in contrast and spectroscopic information, as most of the grains under study are significantly smaller than the foil thickness. High-resolution scanning electron microscopy can usually be used to image the nanocrystalline grain structure. However, quantitative information on grain misorientation using electron backscattered diffraction is not usually possible in cases in which the average grain size is below 150 nm, and this technique is not presently amenable to quantitative chemical mapping with nanoscale (<5 nm) spatial resolution. As such, it is well recognized that there is a paucity of detailed characterization of nanostructured alloys. It is the focus of present research to extend the strength of commercially valuable alloys without sacrificing ductility by engineering nanoscale microstructures or nanostructures. If conventional thermomechanical processing of age-hardenable Al alloys results in a material dominated by dispersions of microscale, solute-rich precipitates, what is the result when SPD is used to engineer nanoscale structures? Furthermore, what relationships would such nanostructures have to the materials properties? We recently reported significant property improvement of a 5083 Al alloy processed by high-pressure torsion (HPT) (composition equivalent to Russian alloy designation 1570) [7] . The alloy had an average grain size of 130 nm and was free of new precipitation. In this study we present a new 7075 Al alloy that expands the known limits of mechanical property performance and provide a comprehensive atomic level investigation of the structure using new high-resolution characterization techniques for both nanostructured alloys. The aerospace-grade 7075 alloy exhibits a yield strength and uniform elongation approaching 1 GPa and 5%, respectively, and both alloys contain a solid solution, free of precipitation, featuring (i) a high density of dislocations, (ii) subnanometre intragranular solute clusters, (iii) two geometries of nanometre-scale intergranular solute structures and (iv) grain sizes tens of nanometres in diameter. Our results demonstrate that this novel architecture offers a design pathway towards a new generation of super-strong materials with new regimes of property-performance space. Materials and mechanical properties We have prepared two types of samples of an aerospace-grade 7075 Al alloy: one by a conventional T6 treatment and the other by HPT engineering. Our stress–strain results, presented in Figures 1a and b , demonstrate an average tensile yield strength and uniform elongation for the HPT alloy (NH-7075) of 0.9775 ± 0.015 GPa and 4.85 ± 0.62%, respectively. The plot in Figure 1a provides a general summary of the fundamental tensile properties of a wide range of metallic Al alloys [6] , [7] , [8] , [9] . Focussing on the NH-7075 alloy, necking is evident when the engineering strain is >5%, and typically resulted in a total elongation to failure of 9%. It is observed that the tendency for postyield strain softening is greatly inhibited in the alloy. These mechanical properties increase the present known limit for the strength of a thermomechanically processed wrought Al alloy prepared by ingot metallurgy and represent approximately twice the strength of a standard T6 age-hardening treatment. 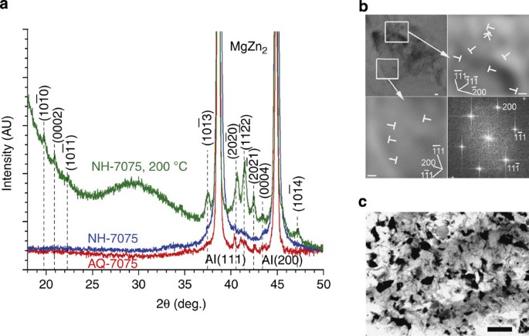Figure 2: X-ray and HRTEM characterization. (a) X-ray diffraction patterns of the quenched 7075 alloy before HPT processing (AQ-7075), HPT processed 7075 Al (NH-7075) and heated NH-7075 to 200 °C (NH-7075, 200 °C) demonstrate that second-phase particles are not detected after HPT processing unless heated to 200 °C, and that the remnant hexagonal MgZn2in the AQ condition is largely dissolved by the processing. The uneven XRD background (such as the broad peak) of the heated sample results from the sample holder. (b) High-resolution TEM reveals a high density of dislocations, marked by 'T' at dislocation cores in the two magnified inverse Fourier transformation images (top left and lower right panels), appearing in both grain interiors and near grain-boundary regions. The fcc solid solution is also observed to be free of precipitation, as revealed by the diffraction pattern in the lower left panel. Scale bar width is 2 nm. (c) Bright-field image of the NH-7075 Al alloy. Scale bar width is 100 nm. Alloy characterization Conventional X-ray diffraction (XRD) analyses, presented in Figure 2a , indicate that the usual minor quantity of second-phase particles remaining after solution treatment was dissolved into the Al matrix by HPT processing. High-resolution TEM (HRTEM) analyses further confirmed the XRD results: the microstructure mostly appears as a continuous solid solution, as demonstrated by the HRTEM images in Figure 2b . Studying the HRTEM images reveals a high density of dislocations within grain interiors and both near and at grain boundaries; dislocation density is ~3.2×10 16 m −2 . The dislocations near and at the grain boundaries have previously been found to form non-equilibrium and small-angle boundaries, respectively [27] , [28] . Bright-field TEM indicates that the present nanostructured 7075 alloy has a 26 nm average grain diameter ( Fig. 2c ). The microstructural assessment exhibits similar features to the previously reported 5083 Al alloy [7] . Figure 2: X-ray and HRTEM characterization. ( a ) X-ray diffraction patterns of the quenched 7075 alloy before HPT processing (AQ-7075), HPT processed 7075 Al (NH-7075) and heated NH-7075 to 200 °C (NH-7075, 200 °C) demonstrate that second-phase particles are not detected after HPT processing unless heated to 200 °C, and that the remnant hexagonal MgZn 2 in the AQ condition is largely dissolved by the processing. The uneven XRD background (such as the broad peak) of the heated sample results from the sample holder. ( b ) High-resolution TEM reveals a high density of dislocations, marked by 'T' at dislocation cores in the two magnified inverse Fourier transformation images (top left and lower right panels), appearing in both grain interiors and near grain-boundary regions. The fcc solid solution is also observed to be free of precipitation, as revealed by the diffraction pattern in the lower left panel. Scale bar width is 2 nm. ( c ) Bright-field image of the NH-7075 Al alloy. Scale bar width is 100 nm. Full size image Novel nanoscale chemical and spatial analysis To investigate the nanostructure and origins for these outstanding properties, we have developed a new atom probe tomography (APT) analysis approach and applied this to these two different alloy systems: Al-Zn-Mg-based 7075 alloy and Al-Mg-Sc-based 5083 alloy. In recent years, APT has been successful in making path-finding structural and chemical measurements by virtue of its atomic resolution and elemental sensitivity [29] , [30] , [31] , [32] , [33] . Advances in instrument technology, improved precision in tomographic reconstruction and the development of application-specific data-processing algorithms have thrust modern APT to the forefront of microscopy [34] , [35] , [36] . The top images in Figures 3a and b present atom maps acquired from the 7075 and 5083 alloy systems after HPT. Inspection of these data gives a qualitative indication of structure and solute aggregation within the alloy. We have developed a novel crystal interface detection method based on analyses of atomic density to reveal the intricate network of grain boundaries; these grain-boundary maps lie below atom maps in Figures 3a and b . Assessment of the 7075 grain dimensions and morphology concurs with the TEM observations ( Fig. 2 ). These images provide clear details of discrete grain-boundary solute enrichment. Specifically, we found that solute atoms aggregate into two basic morphologies on and around select grain boundaries and junctions. We observed point-like 'nodal' and one-dimensional 'lineal' solute arrangements ( Fig. 3b , left). Careful tilting assessments of this tomographic data were conducted to confirm the relative dimensionality of these nanostructural features. The nodal solute nanostructures often occur on triple or higher-order grain-boundary junctions, have a diameter of ~3.7 nm and are observed to occur ~4×10 16 cm −3 . The lineal solute nanostructures extend along grain-boundary vertices, have a length and diameter of ~17.5×~4.4 nm 2 and occur 5×10 16 μm −3 . The lineal nanostructures were also found to occasionally intersect, as seen by the 'V' shape in Figure 4 . 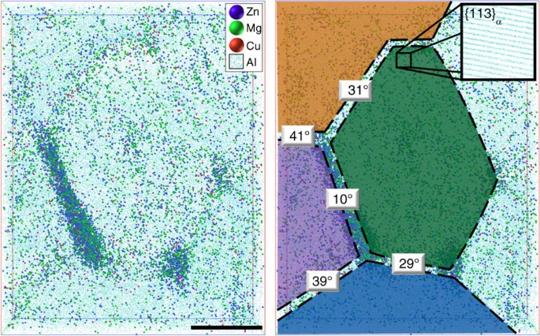Figure 4: Nanoscale texture measurements. Portrait of a grain in the NH-7075 alloy; left, as an atom map, right, with a nanoscale texture map overlaid, indicating the misorientation angle between grains. The lineal solute structure is observed on a grain boundary with a crystal misorientation of 10°. Scale bar width is 5 nm. 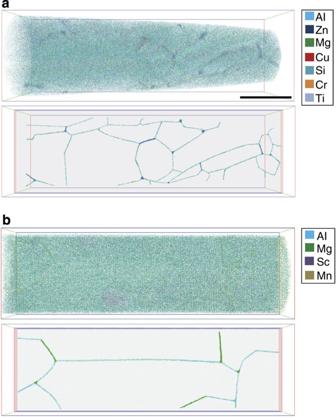Whereas APT analyses of other materials have reported minor global solute segregation to grain boundaries [9] , [37] , [38] , the present findings are significant, as they reveal concentrated and discrete nanometre-sized solute structures at selected grain boundaries. Figure 3: Alloy grain structure. Structural and chemical insights into NH-7075 and NH-5083 alloys from atom probe tomography. The upper images in (a,b) are APT atom maps of specimens of the NH-7075 and NH5083 alloys, respectively. They reveal the first indication of structure and solute aggregation. The lower images reveal the grain-boundary locations in a thin ~1-nm-thick slice of data. Solute is observed to aggregate at certain locations on the boundaries. Scale bar, 50 nm. The atom map in Figure 3c (left) indicates that the intragranular solute is also clustered. Core-linkage clustering algorithm was used to perform a quantitative investigation [34] . 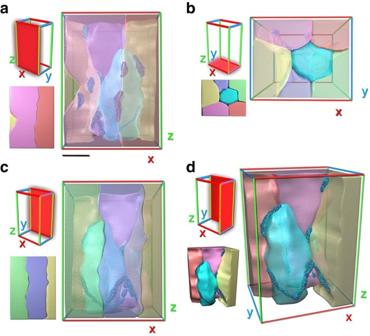Figure 5: Tomographic views of nanostructural architecture in NH-7075 alloy. Line- and node-shaped solute nanostructures strengthen grain-boundary interfaces and junctions. This is communicated through various semitransparent orthographic projections (a–c), and one off-axis, solid, perspective view with certain grains removed to highlight the intergranular nanostructures (d). Scale bar width is 10 nm. Our analysis of cluster number density is provided in Figure 5 . The occurrence of randomly occurring solute clusters was assessed and subtracted from the experimentally observed number density. This analysis reveals that a high concentration of clusters of size 4–7 solute atoms have developed preferentially as the modal cluster type. Figure 3: Alloy grain structure. Structural and chemical insights into NH-7075 and NH-5083 alloys from atom probe tomography. The upper images in ( a , b ) are APT atom maps of specimens of the NH-7075 and NH5083 alloys, respectively. They reveal the first indication of structure and solute aggregation. The lower images reveal the grain-boundary locations in a thin ~1-nm-thick slice of data. Solute is observed to aggregate at certain locations on the boundaries. Scale bar, 50 nm. Full size image Figure 4: Nanoscale texture measurements. Portrait of a grain in the NH-7075 alloy; left, as an atom map, right, with a nanoscale texture map overlaid, indicating the misorientation angle between grains. The lineal solute structure is observed on a grain boundary with a crystal misorientation of 10°. Scale bar width is 5 nm. Full size image Figure 5: Tomographic views of nanostructural architecture in NH-7075 alloy. Line- and node-shaped solute nanostructures strengthen grain-boundary interfaces and junctions. This is communicated through various semitransparent orthographic projections ( a – c ), and one off-axis, solid, perspective view with certain grains removed to highlight the intergranular nanostructures ( d ). Scale bar width is 10 nm. Full size image A more detailed examination of the complex three-dimensional grain-boundary network revealed information on the selective nature of the nodal and lineal solute nanostructures. The right-hand side image of Figure 4 is a nanoscale grain misorientation map derived from APT data: the first published image of this type (see Methods ). An example high-resolution image of the {113} α lattice planes from within the central grain is inset in Figure 4 (right) and other families of crystal planes were similarly observed in this and surrounding grains. Thus, we determined that lineal solute nanostructures were observed exclusively on relatively low-angle grain boundaries, ≤12°. Present statistics on grain misorientation at the region analysed (a half-radius distance from the specimen centre) suggest that ≤50% of boundaries are low angle in nature [39] . Within the two-dimensional grain-boundary surface, lineal structures were observed to follow along the crest of regions of higher grain-boundary curvature. The most obvious characteristic of the sites for solute nodes was that they occurred at grain-boundary junction points, such as triple points. Evidence for this analysis is provided in Figure 5, in which the nanocrystalline topography and grain-boundary solute architecture are imaged in three dimensions. Table 1 provides a summary of the solute balance across the hierarchy of nanostructures in the 7075 alloy (NH-7075); the bulk 7075 alloy composition was determined by metallurgical analysis. At ~2.5 atom % each, Zn and Mg are the two most prominent alloying elements in the 7075 alloy, representing a 1:1 stoichiometric ratio. Combining the information on chemistry and number density, we obtain the relative balance of solute across the observed hierarchy of nanostructural architecture: we find that 38.49% of the solute in the alloy is involved in atomic clustering and most of this is allocated to modal clusters of size 4–7 atoms, with another 51.35%, 8.33% and 1.87% of the solute allocated in the matrix, lines and nodes, respectively. Table 1 Chemical compositions and solute distribution in the NH-7075 alloy. Full size table The 1:1 stoichiometric ratio for Zn and Mg is reflected in the cluster chemistry, but at ~12 times higher concentrations than in the bulk alloy. In addition to containing the highest levels of Cu atoms, these clusters have the greatest concentration of solute of the three nanostructures at ~64 atom %. The nodal and lineal structures exhibit Zn:Mg ratios of approximately 1.5:1, which is similar to compositions traditionally measured for the solute ratio of the metastable η ′ precipitates that are widely cited as the main strengthening element in 7000-series alloys [6] , [40] . The lineal structures are ~5.5 atom % richer in total solute than the nodes, and both the lines and nodes contain elevated levels of Ti. Combining the information on chemistry and number density, we find that 38.49% of the solute in the alloy is involved in atomic clustering and most of this is allocated to the modal clusters of size 4–7 atoms. This compares with only 1.87% of solute in nodes, and with 8.33% in the lineal nanostructures. The remainder (~51%) of the total solute atoms exists in the solid solution in a non-clustered state. We have engineered two crystalline Al alloys to increase the present limits of strength. These alloys feature a nanostructural hierarchy of (i) high dislocation density, (ii) subnanometre intragranular solute clusters, (iii) two geometries of nanometre-scale intergranular nanostructures and (iv) grain sizes tens of nanometres in diameter. In the literature, strength >1 GPa is reached only for Al metallic glasses and for composite Al alloys strengthened by ceramic particles [41] , [42] , [43] . This solute architecture is non-intuitive and, to our knowledge, has not previously been reported. These solute-rich nanostructures are all an intrinsic part of the α-fcc lattice, and none represent a distinct second-phase in the way that, for example, precipitate particles do. We propose that this architecture primarily occurs because of solute-defect (dislocation, point defects and so on) interactions during the nanostructuring process. The high concentration of mobile defects during processing greatly influences the solute dispersion, and the resulting hierarchy reflects an energy landscape in which intragranular solute-clustering and intergranular solute-structuring reactions provide local reductions in free energy. The solute atoms swept to grain boundaries diffuse and populate lineally along grain boundaries and aggregate nodally at grain-boundary junctions. These observations present a fresh perspective to further pursue the origins of material properties and a new starting point for the modelling of strengthening effects. Although it might be considered that the nanocrystalline grain size alone could account for the alloy strength through restriction of dislocation generation and mobility, as described by the Hall–Petch relation, we find, for example, that the parametric constants for the Hall–Petch equation previously determined for pure Al predict a strength of only ~0.27 GPa for the 26 nm average grain size [44] . Similarly, the dissolved (non-clustered) solute will provide very limited conventional solid-solution hardening, considering that a solution-treated 7075 Al alloy with 100% of the solute in the matrix has a strength of 0.145 GPa, whereas only about half (~51%, Fig. 6 ) of the solute remains dissolved in the current sample [8] . Thus, we propose that the near 1 GPa strength and 9% elongation arise from combining the grain size with the observed nanostructural architecture. With regard to the five main deformation mechanisms that might be expected—preexisting dislocation gliding, grain-boundary dislocation emission, grain-boundary sliding, grain rotation and grain-boundary migration—strengthening is expected to occur through the following [24] , [26] , [43] , [45] , [46] , [47] . First, the high density of intragranular solute clusters (comprising ~38% of the total solute) can contribute to significant cluster strengthening, thereby providing effective resistance to slip dislocations, as well as to strain hardening and ductility, by increasing the dislocation storage capability [8] , [48] . Solute clustering has long been reported in conventional coarse-grained or microcrystalline, wrought 7000 Al alloys and linked to strengthening [48] , [49] , [50] , [51] , [52] . For example, alloy hardness can nearly double in the first minute of T6 ageing in a process that cannot be attributed to precipitation [53] , [54] . Furthermore, the dislocations observed within grains may be stabilized by forming Cottrell atmosphere-like solute clustering at the dislocation cores. The strong association of solute to defects in alloys similar to the 7075 composition is well established through positron spectroscopy techniques, and a critical defect concentration has long been established as being essential to the heterogeneous nucleation of metastable precipitates [49] , [50] , [51] , [52] , [55] . The other major architectural features of this solid solution are the intergranular solute nanostructures at grain boundaries. These are expected to provide segregation-based nanocrystal growth stabilization, strengthening interface bond cohesion, and resisting embrittlement and defect generation [23] , [56] . These nodal and lineal solute nanostructures will similarly retard dislocations nucleated at the grain boundaries. Any grain-boundary sliding and rotation will require the breaking or plastic deformation of the intergranular nanostructures, making these energetically more expensive and restricted processes as well. The lineal solute nanostructures on grain boundaries, as observed here, will be available to immobilize grain-boundary dislocations produced during the HPT, and will further strengthen the 7075 alloy. Such dislocations usually exist on non-equilibrium grain boundaries in nanocrystalline metals processed by SPD and are believed to have a significant role in the deformation of nanocrystalline metals [27] , [46] . Room temperature grain-boundary migration under stress has most recently been reported in pure Al with grains of similar size [45] . It is likely that any diffusion-induced migration will be stabilized by the grain-boundary enrichment and that any athermal shear (dislocation-based processes) that would produce the glide of low-angle grain boundaries would encounter similar resistance to that discussed above. 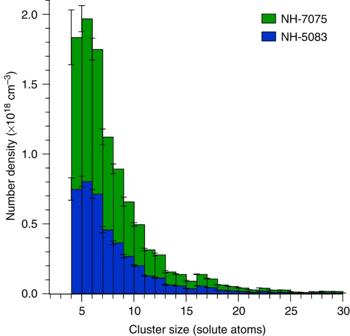Figure 6: Number density of intragranular solute cluster Al alloys. This is shown in green for NH-7075 and in blue for NH-5083. A high concentration of clusters sized 5–9 solute atoms are observed to occur preferentially. The experimentally observed frequency of solute clusters has had the expected random occurrences subtracted (seeMethods); error bars are standard deviation. Figure 6: Number density of intragranular solute cluster Al alloys. This is shown in green for NH-7075 and in blue for NH-5083. A high concentration of clusters sized 5–9 solute atoms are observed to occur preferentially. The experimentally observed frequency of solute clusters has had the expected random occurrences subtracted (see Methods ); error bars are standard deviation. Full size image This nanostructural analysis allows us to contemplate the development of a nanostructural texture, in which information on grain misorientations is combined precisely with information on the solute architecture. The atom probe techniques developed here (for example, Fig. 4 ) will be useful in future development of this concept. The present observations suggest that the hierarchy and architecture of solute have an important influence on nanocrystallinity, grain texture and alloy strengthening. Control of this solute architecture holds promise for development of a new generation of advanced alloys with new regimes of property-performance space. Specimen preparation Commercial 7075 and 5083 Al alloy rods with atomic composition Al-2.55Zn-2.89Mg-0.61Cu-0.11Si-0.10Cr-0.01Ti and Al-6.3Mg-0.1Sc-0.1Mn were solution treated at 480 °C for 5 h and at 380 °C for 2 h, respectively, and then quenched into room-temperature water. The solution-treated rod was machined into 20 mm diameter by 0.8-mm-thick discs. The discs were processed by HPT for 10 revolutions for 7075 and for 20 revolutions for 5083, under a pressure of 6 GPa at room temperature; time elapsed between quench and HPT processing was <20 min. Mechanical property testing Tensile tests were conducted at room temperature at a strain rate of 10 −4 s −1 . The tests were computer controlled, registering temperature, strain and stress. Sample dimensions were accurately measured in our experiments. A laser extensometer, P-50 by Fiedler Optoelectronics, was used to accurately measure the strain. [9] Tensile specimens had 1 mm width and 0.5 mm thickness with a 2-mm-gauge length. The load cell was well calibrated and measurements were determined with a Hottinger Baldwin Messtechnik GmbH firm load sensor with 0.5 tolerance class. Tensile and microscopy specimens were taken from the area at a half-radius distance from the centre of processed discs. Four self-consistent uniaxial tensile tests were completed. The use of miniature specimens has been previously investigated in detail; our studies indicate that, although the strain measurement method and tensile specimen geometry can affect the results, when the strain is accurately measured, the specimen size and geometry only affect the postnecking elongation [57] , [58] . Characterization techniques XRD measurements were taken on a Scintag X-ray diffractometer (Scintag) equipped with a Cu target operating at 1.8 kW. θ – 2θ step scans were taken to record the XRD patterns at room temperature. The scanning step is 0.02° and the scanning rate is 10 s per step. The XRD scanning areas of NH-7075 Al and AQ-7075 Al are dick shaped with a diameter of 20 mm and are therefore comparative. For the NH-7075 at 200 °C, a 4×4 mm 2 sheet of NH-7075 Al was heated to 200 °C in argon atmosphere by differential scanning calorimeter at a heating rate of 5 °C per min, and used for XRD scanning. The XRD patterns of NH-7075 and NH-7075 were recorded at 200 °C upwards in order to see signals of precipitates clearly. The uneven XRD background (such as the broad peak) of the heated sample results from the sample holder. TEM and APT specimens were prepared by standard electropolishing techniques [59] , [60] . Low-energy ion milling was used to clean the TEM foils. TEM was performed on a Philips CM12 (Philips) and a JEOL JEM3000F (JEOL). APT was performed on an Imago LEAP 3000Xsi (Imago). APT acquisitions were performed at a temperature of 20 K, a pulse frequency of 200 kHz, a 25% pulse fraction and a 1% evaporation rate. The reconstruction of APT data was carefully calibrated to crystallographic parameters. Before analysis, low-density erosion of zone and pole lines in the APT data was performed [34] ; a 100 nearest-neighbour (NN) analysis with a 22.5 atoms per nm 3 low-density threshold and 0.5 nm erosion distance was used. Data analysis was performed by using the core-linkage clustering algorithm using atomic point densities [36] . A 26 NN density analysis was used for grain-boundary identification. A 1 NN, 2.5 atoms per nm 3 point density and 0.4-nm d-link core-linkage analysis were used to assess atomic clustering. Taking an atom probe data set and randomly reassigning each atom's element type, according to nominal composition, an identical but chemically homogenous data set could be generated [30] ; the average cluster-size frequencies and standard deviations of 15 homogenized data sets were subtracted from the experimentally observed frequencies to produce Figure 4 . The misorientation of the {001} α plane in each crystal was used to assess texture. When the {001} α was not available, the linear algebraic relationships between a minimum of three non-orthogonal atomic planes were measured and numerically solved for the {001} α plane, with a sum of squares difference error of <1.0°. How to cite this article : Liddicoat, P.V. et al . Nanostructural hierarchy increases the strength of aluminium alloys. Nat. Commun. 1:63 doi: 10.1038/ncomms1062 (2010).